InVERT molding for scalable control of tissue microarchitecture Complex tissues contain multiple cell types that are hierarchically organized within morphologically and functionally distinct compartments. Construction of engineered tissues with optimized tissue architecture has been limited by tissue fabrication techniques, which do not enable versatile microscale organization of multiple cell types in tissues of size adequate for physiological studies and tissue therapies. Here we present an ‘Intaglio-Void/Embed-Relief Topographic molding’ method for microscale organization of many cell types, including induced pluripotent stem cell-derived progeny, within a variety of synthetic and natural extracellular matrices and across tissues of sizes appropriate for in vitro , pre-clinical, and clinical studies. We demonstrate that compartmental placement of non-parenchymal cells relative to primary or induced pluripotent stem cell-derived hepatocytes, compartment microstructure, and cellular composition modulate hepatic functions. Configurations found to sustain physiological function in vitro also result in survival and function in mice for at least 4 weeks, demonstrating the importance of architectural optimization before implantation. Inadequate supply of functional human tissues precludes clinical transplantation for most organ failure patients. Artificial organs and tissues may offer alternatives or bridges to organ transplant. To date, engineered tissues that have been applied clinically (for example, bladder and skin) [1] , [2] contain few cell types and have relatively simple organizational structure. In contrast, construction of complex, highly metabolic tissues such as liver, kidney and heart has seen little success [3] . Complex tissues are spatially organized across functionally and morphologically distinct but interacting compartments (for example, the parenchyma and vasculature). At the microscale, these compartments are often arranged with precise microstructural control in locally repeated functional units (for example, a hepatic cord and associated sinusoid). Such hierarchical positioning of cells within the tissue, or ‘tissue architecture’, ultimately defines the cell–cell contacts and paracrine signalling gradients that drive cellular phenotype and function of each tissue unit, and the collective activity contributed by all units yields large-scale physiological tissue function. Construction of complex engineered tissues requires an understanding of how multi-compartmental tissue architecture dictates whole tissue function both in vitro and after implantation. For such experiments, engineered tissues must also be of adequate mass (contain many repeating microscale tissue units) to generate robust functions measureable by tissue-level experiments and/or to result in a therapeutic outcome. The ability to rapidly organize multiple cell types with microscale precision into units that combine to generate tissues of scalable sizes has remained elusive. To date, several technologies have been developed to position cells at the microscale within engineered tissues, such as dielectrophoresis, photopatterning (including two-photon-based photochemical patterning), cellular bioprinting and topographic molding [4] , [5] , [6] , [7] , [8] , [9] , [10] , [11] , [12] , [13] , [14] , [15] . These technologies enable microscale positioning of cells within 3D engineered tissues, but they often necessitate trade-offs between microscale patterning resolution, tissue size, and/or fabrication time, and they are frequently compatible only with specific biomaterials. Multicellular patterning technologies that are scalable and versatile with regard to biomaterial have the potential to accelerate the development of engineered tissues. Here, we sought to create a platform that (1) enables precise organization of microscale and multi-compartmental tissue structure within tissues of sizes relevant for in vitro , pre-clinical, and clinical studies, and (2) is both material- and cell type-independent and therefore widely biologically applicable. The ‘Intaglio-Void/Embed-Relief Topographic (InVERT) molding’ process described here produced engineered tissues of up to 14 cm in diameter, resulted in viable and high-resolution microstructures organized in distinct compartments in several multicellular patterns, was compatible with fibrin, agarose and polyethylene glycol hydrogel systems and could be used to pattern a variety of cell types, including fragile cell types such as induced pluripotent stem cell-derived hepatocyte-like cells (iPS-Heps), which have not been patternable to date [16] , [17] . We applied our InVERT technology to probe issues relevant to the translation of engineered liver tissue to the clinic. Specifically, crosstalk between hepatocytes and non-parenchymal cells has been implicated in development, physiological homoeostasis, regeneration and disease (for example, malignant transformation) [18] , [19] , [20] , [21] , but systematic dissection of 3D structure–function cellular relationships has proven challenging due to the lack of robust model systems. We used InVERT molding to test whether manipulation of tissue architecture modulates physiological function of primary rat and human hepatocytes or human iPS-Heps in vitro and following implantation in rodents. We found that placement of non-parenchymal cells with respect to primary or iPS-derived hepatocytes and optimization of hepatic compartment microstructure and composition modulates hepatic functions. Additionally, architectural configurations found to sustain hepatic function in in vitro studies also resulted in prolonged survival and physiological function in nude mice after transplantation. These results demonstrate the need for the optimization of microstructural architecture in constructing physiologically robust model systems and engineered tissue therapies. InVERT molding for multi-compartmental cellular patterning We achieved scalable, versatile and rapid 3D multi-compartmental cellular patterning using an InVERT molding protocol ( Fig. 1a ). We first produced topographic substrates containing microscale features and replica molded these substrates using poly(dimethylsiloxane) (PDMS) to create topographic ‘intaglio’ cell-capture substrates with recessed ‘voids’. Cells were added in solution, isolated in the features of the intaglio cell-capture substrate via centrifugation or sedimentation, and then embedded within a 3D hydrogel. Hydrogels containing the patterned cells were removed from the intaglio substrate and inverted, exposing a ‘relief’ (effectively, the inverted intaglio geometry) such that microscale features containing the first cell population projected from the hydrogel. Subsequently, a pre-polymer solution containing a second cell population was loaded on top of the inverted hydrogel (which serves as a secondary mold) and centrifuged into the features of the relief. Polymerization was triggered to trap and encapsulate cells, yielding a 3D hydrogel containing multiple micropatterned cellular compartments. 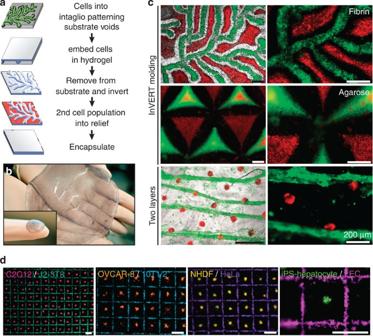Figure 1: Fabrication method and versatility. (a) Process flow diagram for InVERT molding. Seeded cell populations are green (intaglio phase) and red (relief phase). (b) Substrate-based molding produces hydrogels from 1.5 cm- (inset) to 14-cm diameter. Here, size and spacing (800 μm) of cell clusters enables macroscopic visualization after hematoxylin staining. (c) InVERT molding produces multi-compartmental patterning and is compatible with various substrates and materials. Labelled cells (green endothelial cells, calcein-AM; red fibroblasts, calcein red-orange AM) are patterned in fibrin gel using a custom-fabricated branching pattern substrate (top) or in agarose using a substrate molded using a corner cube bike reflector (middle). Substrate-molded cell layers were stacked manually for multilayer patterning (bottom; hepatocyte aggregates, calcein red-orange AM, and endothelial cell cords, green calcein-AM; scale bars, 500 μm unless otherwise denoted). (d) InVERT molding is compatible with many cell types. Mouse C2C12 skeletal myoblasts, mouse J2-3T3 fibroblasts, human ovarian carcinoma cells (OVCAR-8), stromal mouse embryonic fibroblasts (10T1/2), human cervical cancer cells (HeLa), normal human dermal fibroblasts (NHDF) and human iPS-hepatocyte-like cells with liver endothelial cells (TMNK1; LEC) were labelled with calcein dyes and patterned in fibrin gel using InVERT molding (scale bars, 300 μm). Figure 1: Fabrication method and versatility. ( a ) Process flow diagram for InVERT molding. Seeded cell populations are green (intaglio phase) and red (relief phase). ( b ) Substrate-based molding produces hydrogels from 1.5 cm- (inset) to 14-cm diameter. Here, size and spacing (800 μm) of cell clusters enables macroscopic visualization after hematoxylin staining. ( c ) InVERT molding produces multi-compartmental patterning and is compatible with various substrates and materials. Labelled cells (green endothelial cells, calcein-AM; red fibroblasts, calcein red-orange AM) are patterned in fibrin gel using a custom-fabricated branching pattern substrate (top) or in agarose using a substrate molded using a corner cube bike reflector (middle). Substrate-molded cell layers were stacked manually for multilayer patterning (bottom; hepatocyte aggregates, calcein red-orange AM, and endothelial cell cords, green calcein-AM; scale bars, 500 μm unless otherwise denoted). ( d ) InVERT molding is compatible with many cell types. Mouse C2C12 skeletal myoblasts, mouse J2-3T3 fibroblasts, human ovarian carcinoma cells (OVCAR-8), stromal mouse embryonic fibroblasts (10T1/2), human cervical cancer cells (HeLa), normal human dermal fibroblasts (NHDF) and human iPS-hepatocyte-like cells with liver endothelial cells (TMNK1; LEC) were labelled with calcein dyes and patterned in fibrin gel using InVERT molding (scale bars, 300 μm). Full size image To test the scalability and patterning fidelity of substrate-based molding, we created organized arrays of hepatocyte clusters within 3D hydrogels by molding from a PDMS topographic patterning substrate containing pyramidal microwells [22] ( Supplementary Fig. S1a ). We patterned arrays of cellular microstructures within hydrogels to construct tissues with diameters that varied across two orders of magnitude. Sizes of the smallest producible hydrogels were constrained only by the resolution of photopatterning and microfabrication methods. Micropatterned tissues of intermediate size (1.5 cm diameter) were built for subsequent in vitro and mouse studies ( Fig. 1b , inset). Patterned hydrogels of more clinically relevant scales were also achieved (14 cm in diameter; Fig. 1b ). In this large-scale example, cell cluster size and wider spacing allowed for macroscopic detection of cellular patterns after hematoxylin staining, and tissues contained over 24,000 arrayed cellular aggregates. These clusters were patterned in a single molding step (rather than serially). Therefore, cluster spacing could be reduced without altering tissue size and the cellular constitution of all clusters is representative of the cell types included in the initial patterning solution. Scalable gels must also demonstrate fidelity in patterning. We assayed ‘patterning efficiency’, or the percentage of microstructures (here aggregates) successfully patterned in a macroscopic hydrogel upon its removal from the topographic patterning substrate. To detect and count the aggregates present within each hydrogel, we developed a high-throughput, automated large-image scanning and quantitative analysis ( Supplementary Fig. S1a,b ). We assayed patterning efficiency when 1) cells in media were patterned in the topographic microwell substrate, incubated overnight to promote cadherin and adhesion junction formation, and then embedded in a hydrogel, or 2) cells in a pre-polymer solution were added to the topographic mold and trapped immediately by triggering hydrogel polymerization. Patterning efficiency improved with feature size and reached an average of 88±4% (s.e.m.) with pre-aggregation ( Supplementary Fig. S1c ), whereas immediate trapping of cells achieved 97±1% (s.e.m.) for 500 cells per microwell ( Supplementary Fig. S1b ). Thus, substrate-based molding is efficient and compatible with both pre-aggregation and rapid trapping methods. To illustrate the versatility of InVERT molding, we utilized topographic patterning substrates that were either (1) custom-produced using specialized engineering technologies, (2) inexpensive and readily available or (3) high-precision and commercially available. We organized endothelial cells and fibroblasts in four distinct patterns using custom-fabricated substrates with complex topographies (substrates fabricated via computer numerical control micro-milling: Fig. 1c , top; laser engraving: Supplementary Fig. S2 , top; anisotropic etching of silicon [22] : Supplementary Fig. S2 , bottom), a bicycle reflector purchased in a neighbourhood bicycle shop ( Fig. 1c , middle) and a commercially available pyramidal microwell chip (AggreWell, Stem Cell Technologies; Supplementary Fig. S2 ). An ideal patterning technology would be adaptable and modular in nature to enable orthogonal combination with other patterning strategies. We therefore tested whether this method is compatible with previous generation engineering technologies as well as multiple material systems. We demonstrated that micro-organized cell layers produced separately by substrate-based molding could be stacked manually for multilayer patterning ( Fig. 1c , bottom). Additionally, as InVERT molding segregates cellular patterning and encapsulation into distinct steps, this process permits cell encapsulation in a range of natural and synthetic materials with diverse properties, gelation triggers, tunability and general availability and accessibility. For example, InVERT molding could be accomplished using fibrin (gelation by enzymatic polymerization with thrombin: Fig. 1c , top), agarose (gelation by temperature-induced chain entanglements: Fig. 1c , middle) and polyethylene glycol (gelation by external light-based photopolymerization, highly tunable: Supplementary Fig. S2 ). The material in which cells are encapsulated determined pattern maintenance before cellular self-organization. For example, cells remain patterned for weeks without reorganization in non-degradable polyethylene glycol (PEG) gels but began to self-organize over the course of days in highly degradable, low-concentration (for example, 5 mg ml −1 ) fibrin. The time required to perform the InVERT molding inversion step was on the order of minutes, and the time for the entire process depended upon the polymerization time of the material. Additionally, as InVERT molding required no equipment beyond the intaglio topographic substrate and a standard tissue culture centrifuge, parallel and scaled production in a variety of laboratory settings is possible. Together, these results illustrate the versatility of this method for performing rapid multi-compartmental cellular patterning in various orientations and material systems. Finally, to illustrate the applicability of InVERT molding to numerous biological systems, we patterned multiple parenchymal cell types with a variety of non-parenchymal stromal or endothelial cell types. As InVERT molding is based on cell sedimentation or centrifugation, this process is robust regardless of cell-specific physical properties that can impact cell patterning in other systems (for example, size, density, charge). We created multicellular model systems relevant for examining the role of stroma in muscle or cancer biology ( Fig. 1d ; mouse C2C12 skeletal myoblasts with mouse J2-3T3 fibroblasts, human ovarian carcinoma cells (OVCAR-8) with stromal mouse embryonic fibroblasts (10T1/2) and human cervical cancer cells (HeLa) with stromal normal human dermal fibroblasts (NHDF)). As InVERT molding does not exert forces on cells that would not otherwise be experienced during routine tissue culture, we hypothesized that this technique would be extensible to ‘sensitive’ cell types that have not been not been patterned successfully using other methods (for example, iPS-derived cells). Towards this end, we used InVERT molding to pattern human iPS-Heps with liver endothelial cells (TMNK1; LEC; Fig. 1d ). By visualizing molded cells in all panels of Fig. 1 with calcein viability dyes, we observed that most cells examined retained intact plasma membranes ( Fig. 1 ; all panels with fluorescently labelled cells). Quantitative live–dead analysis using calcein-AM (live, green) and ethidium homodimer (red) demonstrated that the percentage of living cells was cell-type-dependent and reached 99±1% (s.e.m. ; Supplementary Fig. S3 ). These results demonstrate that cells, despite physical properties or origin, can be patterned, encapsulated, and demolded using the InVERT molding technique. InVERT molding could thus be useful in a variety of biological model systems and engineered tissue applications. Multicellular microorganization across distinct compartments We next sought to further characterize the microscale organization of distinct cellular compartments in 3D engineered tissue constructed using InVERT molding. We used InVERT molding to encase microorganized hepatic aggregates (red; calcein red-orange AM) within an endothelial cell lattice (green; calcein-AM) in a hydrogel ( Fig. 2a ). This process produced 1.5-cm diameter hydrogels containing ~1,000 hepatic aggregates ( Fig. 2b , top left; each aggregate composed of ~125 cells). Opaque oblique and cross-sectional renderings of stacked multiphoton images demonstrated that the cellular microstructures in both compartments spanned a thickness of ~130 μm ( z direction; Fig. 2b , middle and bottom). Unlike systems that create multicellular patterning by stacking separate layers, hepatic and endothelial compartments exhibit substantial z -plane overlap in the InVERT molded tissue ( Fig. 2b , middle). Compartments do not overlap in the x–y plane ( Fig. 2b , middle). z -plane overlap can be reduced or removed by altering cell concentration in each compartment ( Fig. 2b , bottom left). 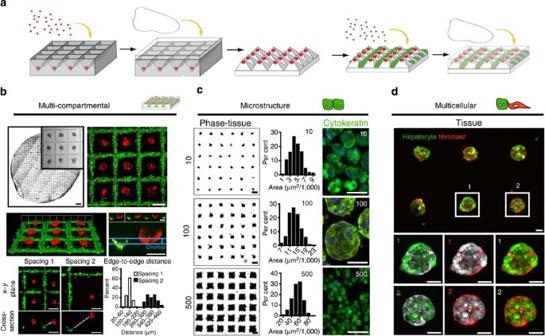Figure 2: Multi-level and multicellular microorganization can be controlled across and within distinct compartments. (a) Hepatic aggregates (red) were embedded within an endothelial lattice (green) using InveRT molding. (b) Each 1.5-cm diameter hydrogel contained ~1,000 aggregates (top left, representative phase images; scale bar, 1 mm; inset, 200 μm). Hepatic aggregates (red, calcein red-orange AM) were patterned within the endothelial lattice (green; calcein-AM, top right; scale bar, 200 μm). 3D patterning is evident from opaque oblique and cross-sectional rendering of stacked multiphoton images (middle left; grid scale bar, 127 μm). A single cross-section slice reveals overlap between populations in thezplane (blue lines) but no overlap in thex–yplane (middle right). Altering cell-seeding density of J2 fibroblast aggregates and liver endothelial cells can eliminate overlap (bottom left; scale bars, 110 μm). Edge-to-edge distance (dotted white line) between cellular compartments followed distinct Poisson distributions for different spacings (bottom right) and was 116±25 μm s.d. and 366±52 μm (s.d.), respectively. (c) An average of 10–500 hepatocytes were seeded per microwell. Resultant aggregates were either encapsulated in hydrogels or removed for immunostaining analysis. Aggregates encapsulated in hydrogels (left; scale bar, 200 μm) exhibit Poisson distribution (centre; average cross-sectional area of 50±15 × 102μm2, 145±28 × 102μm2and 590±110 × 102μm2(s.d.) for 10, 100 and 500 cell aggregates, respectively). Cytokeratin immunostaining of isolated aggregates reveals distinct morphology across aggregate sizes (right, scale bar 50 μm). (d) Multiphoton imaging of hydrogels with patterned aggregates containing both hepatocytes and J2 fibroblasts demonstrates that fibroblasts were dispersed throughout each hepatic aggregate (fibroblasts, mCherry; hepatocytes, calcein-AM; scale bar, 50 μm). Representative aggregates show fibroblasts located at both the edges and center of the aggregates (bottom). Figure 2: Multi-level and multicellular microorganization can be controlled across and within distinct compartments. ( a ) Hepatic aggregates (red) were embedded within an endothelial lattice (green) using InveRT molding. ( b ) Each 1.5-cm diameter hydrogel contained ~1,000 aggregates (top left, representative phase images; scale bar, 1 mm; inset, 200 μm). Hepatic aggregates (red, calcein red-orange AM) were patterned within the endothelial lattice (green; calcein-AM, top right; scale bar, 200 μm). 3D patterning is evident from opaque oblique and cross-sectional rendering of stacked multiphoton images (middle left; grid scale bar, 127 μm). A single cross-section slice reveals overlap between populations in the z plane (blue lines) but no overlap in the x–y plane (middle right). Altering cell-seeding density of J2 fibroblast aggregates and liver endothelial cells can eliminate overlap (bottom left; scale bars, 110 μm). Edge-to-edge distance (dotted white line) between cellular compartments followed distinct Poisson distributions for different spacings (bottom right) and was 116±25 μm s.d. and 366±52 μm (s.d. ), respectively. ( c ) An average of 10–500 hepatocytes were seeded per microwell. Resultant aggregates were either encapsulated in hydrogels or removed for immunostaining analysis. Aggregates encapsulated in hydrogels (left; scale bar, 200 μm) exhibit Poisson distribution (centre; average cross-sectional area of 50±15 × 10 2 μm 2 , 145±28 × 10 2 μm 2 and 590±110 × 10 2 μm 2 (s.d.) for 10, 100 and 500 cell aggregates, respectively). Cytokeratin immunostaining of isolated aggregates reveals distinct morphology across aggregate sizes (right, scale bar 50 μm). ( d ) Multiphoton imaging of hydrogels with patterned aggregates containing both hepatocytes and J2 fibroblasts demonstrates that fibroblasts were dispersed throughout each hepatic aggregate (fibroblasts, mCherry; hepatocytes, calcein-AM; scale bar, 50 μm). Representative aggregates show fibroblasts located at both the edges and center of the aggregates (bottom). Full size image Different signalling activators and inhibitors are known to act across varying distances, but relative contributions of specific factors responsible for such differences have not been elucidated due to in vivo model system complexity [23] , [24] , [25] . A 3D system that precisely places two cell populations at varying distances could enable previously impossible in vitro interrogation of distance-reliant multicellular interactions. Here, edge-to-edge spacing between tissue compartments was controlled by altering the topography of the intaglio-patterning substrate used for InVERT molding ( Fig. 2b , bottom left). The distance between each cellular aggregate and its closest endothelial neighbour ( Fig. 2b , bottom right; dotted white lines) followed non-overlapping Poisson distribution for different spacing configurations ( Fig. 2b , bottom). Average edge-to-edge distances were 116±2 μm (s.e.m.) and 366±4 μm, respectively (s.e.m., P <0.01, Student’s t -test), which are relevant for studying intercellular communication via soluble signals [23] , [26] . Together, these results demonstrate the ability to control inter-compartmental spacing and microorganization of multiple cell types across distinct tissue compartments using InVERT molding. Altering microstructure and composition within a compartment Complex tissues are hierarchically organized such that each tissue compartment is further organized at both the microstructural and multicellular level. Therefore, we tested whether InVERT molding could be applied to fine-tune the composition of microtissue units within a given compartment. Specifically, we refined the hepatic compartment produced during the initial Intaglio-Void-Embed portion of the InVERT molding protocol without adding a second cell population (‘relief’ phase). Primary rat hepatocytes were seeded in patterning substrates at densities of 10–500 cells per microwell and incubated overnight. The combined use of oblique microwell side-walls and complete surface tiling resulted in collection of all cells within a defined volume followed by aggregate formation. Following aggregate encapsulation, hydrogels were imaged to quantify the sizes of resulting microstructures using our automated platform ( Supplementary Fig. S1 ). Varying hepatocyte seeding density produced distinct Poisson distributions of aggregate size ( Fig. 2c ). Aggregates formed from 10, 100 and 500 cells per microwell had an average cross-sectional area of 50±1 × 10 2 μm 2 , 145±2 × 10 2 μm 2 and 590±5 × 10 2 μm 2 (s.e.m. ), respectively. Immunohistological analysis of hepatocyte aggregates demonstrated distinct morphologies were obtained according to the number of cells seeded. Specifically, aggregates created from 10 or 100 hepatocytes contained intact intercellular junctions, whereas cells in larger aggregates remained isolated and dispersed ( Fig. 2c , right; cytokeratin, green. Note: scale bar is 50 μm for all histological images). To further modulate multicellular composition in a given micropatterned cellular compartment, we generated hydrogel-encapsulated ‘heteroaggregates’ by seeding a mixed population of hepatocytes and mural J2 fibroblasts (‘fibroblasts’) and encapsulating resulting aggregates in hydrogels ( Fig. 2d ). Multiphoton imaging of these hydrogels demonstrated that fibroblasts expressing mCherry (red) were intercalated throughout the hepatic aggregates (green, calcein-AM–labelled, Fig. 2d ). Taken together, these results demonstrate the ability to modulate both microstructure and multicellular composition of units within a given tissue compartment using InVERT molding. Organization of endothelial cells impacts tissue function We next sought to evaluate the biological applicability of InVERT molding. We tested whether varied positioning of an endothelial cell compartment would affect hepatic parenchymal tissue function, as endothelial cells can modulate parenchymal functions in both health and disease via the release of ‘angiocrine’ factors [20] , [27] . Liver sinusoidal endothelial cells (green) were patterned either directly into microwells adjacent to hepatic aggregates (red; ‘juxtaposed’ conformation) before hydrogel encapsulation or in a compartmentally distinct cellular lattice (‘paracrine’ conformation) via InVERT molding ( Fig. 3a , left). Cell numbers of each individual population were held constant in all hydrogels. Patterning endothelial cells in a paracrine conformation enhanced albumin secretion, a surrogate measure of hepatic function, over twofold compared with patterning endothelial cells in juxtaposed conformation ( Fig. 3a , center). Hepatic aggregates patterned without endothelial cells exhibited similar functional activity to those patterned in ‘paracrine’ conformation ( Supplementary Fig. S4 ). These findings demonstrate that varying the microorganization of the endothelial compartment can alter the hepatic functions of engineered tissues. 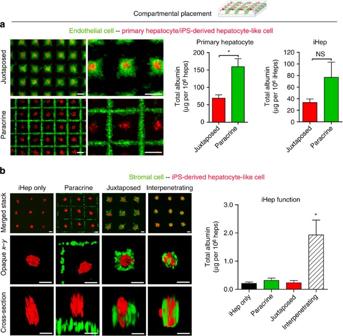Figure 3: Multi-compartmental placement dictates hepatic tissue function. (a) Liver sinusoidal endothelial cells (green) were patterned in ‘juxtaposed’, or compartmentally distinct ‘paracrine’ conformations relative to hepatic aggregates using InVERT molding (scale bar, 200 μm). Paracrine configurations for primary hepatic aggregates and liver endothelial cells yield significantly greater albumin secretion than juxtaposed configurations (P=0.0087, error bars denote s.e.m.,n=5 and 6 and 160±56 and 69±22 μg per 106hepatocytes (s.d.) for each respective group, Mann–Whitney test *P<0.05), and similar trends were observed for iPS-Hep aggregates though this data was not significant (P=0.3500, error bars denote s.e.m.,n=3 for both groups, 77±45 and 33±11 ng per 106hepatocytes (s.d.) for paracrine and juxtaposed groups, respectively; Mann–Whitney test). (b) Stromal cells (green) were patterned either in paracrine, juxtaposed’ or ‘interpenetrating’ conformation relative to iPS-hepatocyte-like cells using InVERT moudling (scale bars, 200 μm). Interpenetrating configurations yield higher albumin secretion relative to other conformations (*P<0.05,P=0.0250, error bars denote s.e.m.,n=5, 4, 6, 6 and 0.2±0.1, 0.3±0.2, 0.2±0.2, 1.9±1.3 μg per 106iHeps (s.d.) for each respective group; one-way ANOVA with Tukeypost-hoctest). Figure 3: Multi-compartmental placement dictates hepatic tissue function. ( a ) Liver sinusoidal endothelial cells (green) were patterned in ‘juxtaposed’, or compartmentally distinct ‘paracrine’ conformations relative to hepatic aggregates using InVERT molding (scale bar, 200 μm). Paracrine configurations for primary hepatic aggregates and liver endothelial cells yield significantly greater albumin secretion than juxtaposed configurations ( P =0.0087, error bars denote s.e.m., n =5 and 6 and 160±56 and 69±22 μg per 10 6 hepatocytes (s.d.) for each respective group, Mann–Whitney test * P <0.05), and similar trends were observed for iPS-Hep aggregates though this data was not significant ( P =0.3500, error bars denote s.e.m., n =3 for both groups, 77±45 and 33±11 ng per 10 6 hepatocytes (s.d.) for paracrine and juxtaposed groups, respectively; Mann–Whitney test). ( b ) Stromal cells (green) were patterned either in paracrine, juxtaposed’ or ‘interpenetrating’ conformation relative to iPS-hepatocyte-like cells using InVERT moudling (scale bars, 200 μm). Interpenetrating configurations yield higher albumin secretion relative to other conformations (* P <0.05, P =0.0250, error bars denote s.e.m., n =5, 4, 6, 6 and 0.2±0.1, 0.3±0.2, 0.2±0.2, 1.9±1.3 μg per 10 6 iHeps (s.d.) for each respective group; one-way ANOVA with Tukey post-hoc test). Full size image Organization of stromal compartment alters iPS-Hep function Human iPS cells have potential for use in in vitro model systems as well as translatable human cell-based tissue therapies. In the context of the liver, human hepatocyte-like cells (iPS-Heps) have recently been generated from iPS and used in 2D model systems [16] , [17] , but optimal architectural parameters for organizing these cells in a 3D setting have not been elucidated. We sought to use InVERT molding to dissect multicellular geometrical conformations necessary for the maintenance of hepatic iPS-Hep function. We first tested whether patterning of liver sinusoidal endothelial cells in juxtaposed or paracrine conformation modulates iPS-Hep function and found that, similar to primary hepatocytes, patterning in paracrine conformation trended towards enhanced hepatic function, though these results were not significant. Next, iPS-Heps (red) were seeded at a density of 100 cells per microwell, and stromal fibroblasts (green; constant number for all hydrogels) were patterned in a compartmentally distinct lattice (‘paracrine’ conformation), adjacent to iPS-Hep aggregates that had already compacted (‘juxtaposed’ conformation) or directly into microwells with iPS-Heps to create a heteroaggregate (‘interpenetrating’ conformation) ( Fig. 3b ). Direct patterning of stromal cells to form heteroaggregates (interpenetrating’) resulted in optimal hepatic function ( Fig. 3b ), suggesting that local paracrine or direct contact signals with the stroma are important for the function or maturation of iPS-Heps ( Fig. 3b ). Microstructure and multicellular composition impact function In addition to patterning cells between compartments, we used InVERT molding to test whether alterations in the microstructure and multicellular composition of aggregates within the parenchymal compartment might further impact engineered liver tissue function. We altered parenchymal compartment microstructure by creating hydrogels with 10, 100 or 500 hepatocytes per homotypic aggregate. Hepatic albumin secretion per hepatocyte was dependent on the number of cells plated per microwell, and function began to decline by 4 days after seeding in each case ( Fig. 4a ). After 4 days in culture, microtissues containing 100 hepatocytes per aggregate produced 14-fold greater albumin per hepatocyte than those formed by seeding 500 hepatocytes per aggregate ( Fig. 4a ). These results were notable given the morphological differences between aggregates containing 100 or 500 hepatocytes ( Fig. 2c ). We hypothesized that additional control of multicellular composition within the parenchymal compartment would further stabilize tissue function, as has been shown previously in other model systems [21] , [28] . Indeed, the inclusion of hepatocyte–fibroblast heteroaggregates in patterned tissues resulted in significant enhancement and prolongation of hepatic functions to at least 12 days in a dose-dependent manner ( Fig. 4b ). These results demonstrated that, in addition to relative compartmental location, the microstructure and multicellular composition of the units within a given compartment (here, the parenchymal compartment) significantly impacts engineered tissue function. Together, our results demonstrate the biological importance of hierarchical architectural optimization when constructing engineered tissues. 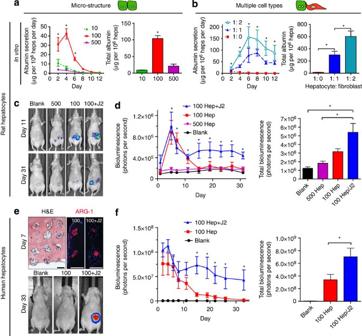Figure 4: Optimization of tissue architecture modulates hepatic functionin vitroandin vivo. (a) The number of hepatocytes per aggregate (10–500) resulted in distinct hepatic tissue functionin vitro(*P<0.05, error bars denote s.e.m.,n=4, 3, 3 and total albumin of 9±2, 104±12, 21±9 (s.d.) for each respective group, Kruskal–Wallace test). (b) Addition of J2 fibroblasts to hepatic aggregates in hydrogels sustained (left) and improved cumulative (right) hepatic functions in a dose-dependent mannerin vitro(100 hepatocytes per aggregate+fibroblasts at 1:0, 1:1, 1:2 hepatocytes:fibroblast, *P<0.05, error bars denote s.e.m.,n=5, 5, 4 and total albumin of 15±4, 300±132, 602±179 μg per 106hepatocytes (s.d.) for each respective group, one-way ANOVA with Tukeypost-hoctest). (c) Representative bioluminescence images of nude mice that received patterned tissue containing no cells (‘Blank’), 500 rat primary hepatocytes per aggregate (‘500’), 100 hepatocytes per aggregate (‘100’), or 100 hepatocytes+J2 fibroblasts per aggregate (‘100+J2’) implanted in the intraperitoneal space. (d) Optimalin vitrotissue configurations result in sustained hepatic functions to over 4 weeks following implantation (*P<0.05, error bars denote s.e.m.,n=3, 4, 5, 6 and total bioluminescence of 1.2e6±0.3e6, 1.8e6±0.5e6, 3.2e6±0.8e6, 5.4e6±2.3e6 (s.d.) for each respective group, Kruskal–Wallace test with Dunn’s Multiple Comparisonpost-hoctest). (e) Representative histological images of patterned tissues containing 100 cryopreserved human hepatocytes per aggregate with or without J2 fibroblasts (‘100’ or ‘100+J2’) that were extracted 7 days after intraperitoneal implantation in nude mice. Patterned arrays of aggregates (left, hematoxylin and eosin) that contained arginase-1-positive hepatocytes (right, ARG-1, red) were identified in all animals with cellular implants (scale bars, 100 μm). (f) The addition of fibroblasts sustained human hepatic function for at least 4 weeks (*P<0.05, error bars denote s.e.m.,n=4, 6, 6 and total bioluminescence of 0.0e8±0.0e8, 3.4e8±2.1e8, 7.0e8±3.3e8 (s.d.) for each respective group, Mann–Whitney test, ‘blank’ excluded from statistical analysis). Figure 4: Optimization of tissue architecture modulates hepatic function in vitro and in vivo . ( a ) The number of hepatocytes per aggregate (10–500) resulted in distinct hepatic tissue function in vitro (* P <0.05, error bars denote s.e.m., n =4, 3, 3 and total albumin of 9±2, 104±12, 21±9 (s.d.) for each respective group, Kruskal–Wallace test). ( b ) Addition of J2 fibroblasts to hepatic aggregates in hydrogels sustained (left) and improved cumulative (right) hepatic functions in a dose-dependent manner in vitro (100 hepatocytes per aggregate+fibroblasts at 1:0, 1:1, 1:2 hepatocytes:fibroblast, * P <0.05, error bars denote s.e.m., n =5, 5, 4 and total albumin of 15±4, 300±132, 602±179 μg per 10 6 hepatocytes (s.d.) for each respective group, one-way ANOVA with Tukey post-hoc test). ( c ) Representative bioluminescence images of nude mice that received patterned tissue containing no cells (‘Blank’), 500 rat primary hepatocytes per aggregate (‘500’), 100 hepatocytes per aggregate (‘100’), or 100 hepatocytes+J2 fibroblasts per aggregate (‘100+J2’) implanted in the intraperitoneal space. ( d ) Optimal in vitro tissue configurations result in sustained hepatic functions to over 4 weeks following implantation (* P <0.05, error bars denote s.e.m., n =3, 4, 5, 6 and total bioluminescence of 1.2e6±0.3e6, 1.8e6±0.5e6, 3.2e6±0.8e6, 5.4e6±2.3e6 (s.d.) for each respective group, Kruskal–Wallace test with Dunn’s Multiple Comparison post-hoc test). ( e ) Representative histological images of patterned tissues containing 100 cryopreserved human hepatocytes per aggregate with or without J2 fibroblasts (‘100’ or ‘100+J2’) that were extracted 7 days after intraperitoneal implantation in nude mice. Patterned arrays of aggregates (left, hematoxylin and eosin) that contained arginase-1-positive hepatocytes (right, ARG-1, red) were identified in all animals with cellular implants (scale bars, 100 μm). ( f ) The addition of fibroblasts sustained human hepatic function for at least 4 weeks (* P <0.05, error bars denote s.e.m., n =4, 6, 6 and total bioluminescence of 0.0e8±0.0e8, 3.4e8±2.1e8, 7.0e8±3.3e8 (s.d.) for each respective group, Mann–Whitney test, ‘blank’ excluded from statistical analysis). Full size image Microorganization modulates tissue function in vivo Successful clinical translation of complex engineered tissue will require the maintenance of highly functional parenchyma following tissue implantation. We hypothesized that tissue conformations that resulted in sustain tissue function in vitro would also sustain tissue function in vivo . To test this hypothesis, we transduced primary rat hepatocytes with a lentivirus in which a modified albumin promoter [29] drives the expression of firefly luciferase, created patterned engineered liver tissues according to the specifications that produced differing hepatic functions in our in vitro studies (that is, 100 versus 500 hepatocytes per aggregate and ± fibroblast in aggregates with 100 hepatocytes), implanted the resulting tissues in the intraperitoneal (IP) space of nude mice, and monitored bioluminescence of the grafted tissues. Consistent with our in vitro observations, the number of hepatocytes per aggregate augmented tissue function over fourfold by 5 days after implantation and was optimal at 100 hepatocytes per aggregate ( Fig. 4c ). The addition of fibroblasts enhanced hepatic function 2–3 fold starting at day 15 and maintained albumin secretion for at least 4 weeks after implantation ( Fig. 4d ). We hypothesized that as this method enables patterning of delicate cell types, patterned tissues containing clinically relevant, cryopreserved human hepatocytes would survive and function in vitro and in vivo. We found that tissues containing human hepatocytes that contained fibroblasts exhibited secreted over 33-fold greater albumin by day 6 compared with those containing only hepatocytes in vitro ( Supplementary Fig. S5 ). Human hepatocytes expressing luciferase under the control of a modified albumin promoter were then patterned in tissues that contained heteroaggregates of 100 hepatocytes ± fibroblasts, and implanted in the IP space of nude mice. Histological examination of explanted human hepatocyte tissues demonstrated that patterned arrays of hepatic aggregates were generally retained at 1 week after implantation ( Fig. 4e , left, hematoxylin and eosin). Arginase-1 (ARG-1) immunostaining identified human hepatocytes within the aggregates, which self-sorted to the center of each aggregate in tissues that contained fibroblasts by 1 week after implantation ( Fig. 4e , right). Gross examination upon resection of engineered tissues at day 7 demonstrated that 74% of implants adhered to host tissue (14 of 19 tissues, Supplementary Fig. S6 ), and Ter-119-positive red blood cells were identified in these explants. The average distance from Ter-119-positive blood and the nearest ARG-1-positive-hepatic aggregate was 119±32 μm (s.e.m. ; Supplementary Fig. S6 ), suggesting that nutrient transport in the system occurred via diffusion from de novo vessels derived from the host to the hepatic aggregates. Similar to rat hepatic tissues, hepatic function in aggregates with 100 hepatocytes was sustained by the presence of fibroblasts ( Fig. 4f ). Thus, optimal cellular architectures that sustained hepatic functions in vitro to day 12 also resulted in superior physiological tissue function for at least 4 weeks after transplantation in pre-clinical animal models. Our InVERT molding platform rapidly yields high-resolution multicellular microstructures that can be patterned in distinct compartments in 3D hydrogels. This process offers numerous advantages over previous systems. Substrate-based molding is scalable and can produce tissue sizes ranging over two orders of magnitude without significantly altering microstructure, resolution or assembly time. This process can be used to pattern either ‘pre-aggregated’ cells with established intercellular junctions necessary for normal physiological functions in most tissues, or to immediately ‘trap’ cells, akin to other patterning technologies. Importantly, this method is compatible with customizable topographic patterning substrates and material systems employed in specialized engineering and biomaterials research laboratories as well as with materials commonly found in basic biological laboratories. Further, InVERT molding is based on gravity or centrifugation-enhanced sedimentation and therefore appears to cause minimal cell damage, even to otherwise sensitive cell types. As the InVERT molding process also does not require tedious manual alignment of cell layers and can be parallelized, production of patterned hydrogels is rapid. Finally, InVERT molding enables the multi-level hierarchical optimization of tissue structure both within and between cellular compartments. Together, these features of InVERT molding uniquely enable large-scale biological studies that probe how complex tissue structure dictates cellular behaviour. Vascular endothelial and stromal cells have important roles in tissue development, homoeostasis and function in health and disease [18] , [19] , [20] , [27] , [30] . Here, we found that the structural organization of liver endothelial and stromal cells modulates the degree to which they support and stabilize hepatic parenchyma. For endothelial cells, possible mechanisms include hepatic interaction with inhibitory endothelial cell surface molecules (for example, cadherin), extracellular matrix molecules or short-range or matrix-sequestered soluble factors in juxtaposed but not paracrine conformation. For tissues containing stromal cells and iPS-Heps, interactions likely occur via local paracrine or direct contact signals, as intimate contact between iPS-Heps and stromal cells is required throughout the entire aggregate (‘interpenetrating’ conformation). It is possible that short-range molecular mediators of interactions between adult primary hepatocytes and J2 stromal cells, such as decorin and truncated-cadherin could impact iPS-Hep function [31] , [32] . Together, our studies suggest that InVERT molding may be useful for the methodical dissection of the relative contribution of multi-factorial signals (for example, cell contact, paracrine signals, extracellular matrix) on the differentiation state or signalling activity of stem cell progeny or tissue organoids. Numerous techniques have been used to create hepatic spheroids with intact intercellular contacts, structural polarity, functional bile canaliculi and hepatic functions [33] , [34] , [35] , [36] , [37] , [38] . Our pyramidal microwell-based patterning system improves cell-capture efficiency due to lack of dead space between microwells, allows precise control of cell number seeded per microwell and resultant aggregate diameter and prevents aggregate fusion and loss over time by capturing aggregates at defined locations in 3D gels. This progress allowed us to demonstrate that structural refinement of engineered tissues must be performed not only between but also within tissue compartments. Recent studies have shown that the inclusion of multiple cell types or further microvascular patterning in engineered tissues can improve survival and/or function after engraftment [29] , [39] , [40] , [41] . To our knowledge, ours is the first study to demonstrate the importance of optimizing multicellular parenchymal structure before implantation to maximize tissue function after transplant. Although we demonstrate this principle using both clinically relevant iPS-Heps and cryopreserved human hepatocytes, ultimate application in clinical therapy will require additional advances. For example, z -direction thickness of InVERT molded tissue is limited by nutrient diffusion, as tissues do not contain conduits for fluid flow, and thus upon implantation tissues relies on vascularization by the host. Combination of the InVERT system with other technologies that improve graft vascularization [13] , [42] could enable construction of thicker tissues and enhanced function of metabolically active hepatocytes. Additionally, it will be necessary to demonstrate long-term survival of grafted cells and rescue of missing liver functions in genetic liver disease or acute liver failure model systems. The InVERT molding platform described here may impact the creation of model systems for studying basic biology as well as lead to the development of specific architectural ‘design specifications’ for the construction of clinically relevant engineered tissue therapies. This technology could be useful in diverse fields ranging from regenerative medicine to cancer pathogenesis. Microfabrication of intaglio-patterning substrates Square pyramidal microwells were fabricated as described previously [22] or purchased (AggreWell, Stem Cell Technologies; 400 or 800 μm side-wall dimension of each square pyramidal micro-well). For branching network substrates, patterns were first generated by computer numerical control milling (Taig DSLS3000) in high-temperature epoxy (Conapoxy FR1080, Cytec) and then cast in PDMS. For spiral substrates, patterns were laser-engraved in acrylic (Versalaser VLS3.50, Universal Laser Systems) and then cast in PDMS. Cell culture and labelling See Supplementary Methods . Hydrogel materials For agarose gels, ultra-pure low-melting point agarose (Invitrogen) was dissolved in DMEM (2% w/v). Liquid agarose solution was kept in a water bath at 37 °C until time of cell encapsulation and polymerization, at which point it was pipetted over patterned cells in the intaglio substrate and cooled at 4 °C to initiate gelation. Fibrin hydrogels were prepared by adding human thrombin (Sigma; 1.25 U ml −1 final concentration) to bovine fibrinogen (Sigma; 20 mg ml −1 final concentration) at the time of polymerization or by suspending cells in fibrinogen at the appropriate concentration, centrifuging into the secondary relief mold and polymerizing via the addition of thrombin. For PEG hydrogels, cells were suspended in PEG pre-polymer solution, centrifuged into the secondary relief PEG material template, and then exposed to UV light from a spot-curing system with collimating lens (320–390 nm, 90 mW cm −2 , 30 s, EXFO lite). PEG pre-polymer solution was composed of PEG-diacrylate (20 kDa at 10% (w/v); Laysan Bio) and 0.1% (w/v) Irgacure 2959 (Ciba). Fabrication of micropatterned engineered tissues For InVERT molding, the first cell population was either centrifuged or gravity settled (for hydrogels >10 cm in diameter) into the recessed features of the intaglio-patterning substrate. A silicon gasket defining the x–y–z dimensions of the resultant hydrogel was placed over the cells arrayed in the patterning substrate. For ‘pre-aggregation’-based encapsulation, cells were incubated overnight. The following day, the hydrogel material was pipetted over the cells and polymerized. For ‘immediate trapping’, cells were spun into the patterning substrate directly in pre-polymer solution and then trapped in place by polymerization. Molded 3D hydrogels containing the first patterned cell type were removed from the intaglio substrate and inverted, exposing ‘relief’ features in the molded hydrogel. The inverted relief gel was placed into a second gasket system, and a new cell population in pre-polymer solution was centrifuged into place. Polymerization was triggered to entrap cells, resulting in the formation of a single hydrogel containing two distinct and micro-organized cellular compartments. For studies demonstrating the application of InVERT molding with many cell types ( Fig. 1d ), the first cell type was seeded into ‘intaglio’ microwell templates (microwell side-wall dimensions 400 μm at a concentration of 100 cells per microwell) before material encapsulation. The second ‘relief’ cell type was patterned using InVERT molding such that final cell ratio was 1:0.5 for cell type 1:cell type 2. For studies of hepatocyte and J2 fibroblast microorganization, 10–500 hepatocytes per microwell and corresponding J2 fibroblasts at ratios 1: 1 or 1: 2 were centrifuged into microwell templates (microwell side-wall dimensions 400 μm). The following day, resultant aggregates were encapsulated in either agarose or fibrin hydrogels. For studies of multi-compartmental organization, 100 primary rat or iPS-Heps and 25 J2 fibroblasts were patterned per microwell, incubated overnight and then encapsulated in fibrin. Liver endothelial cells were then patterned using InVERT molding in either juxtaposed or paracrine conformations at a final concentration of two endothelial cells per hepatocyte. For multi-compartmental studies with iPS-Heps and stromal cells only, 100 iPS-Heps were patterned per well and J2 fibroblasts were patterned in various conformations at a ratio of 1: 1 iPS-Hep:J2 fibroblast. For studies in which inter-compartmental distance was varied, 100 J2 fibroblasts expressing GFP were patterned in microwells with side-wall dimensions of 400 or 800 μm. Liver endothelial cells were then patterned using InVERT molding, and hydrogels were imaged using live imaging methods described below. For hydrogels of 14 cm diameter, J2 fibroblasts were fixed and stained with hematoxylin before encapsulation for macroscopic visualization. A total of 800 fibroblasts per well were gravity settled into a 14-cm diameter patterning substrate containing microwells with side-wall dimensions of 800 μm. Cells were encapsulated in fibrin gel and imaged with a Nikon digital SLR camera. For biological experimentation, a quality control step was introduced during manufacturing at the time of demolding such that gels with <80% patterning efficiency were discarded immediately after demolding and before further biological study. Thus, although the same number of gels was initially patterned per group, biological experiments sometimes had groups with slightly different ‘n’. In contrast, for engineering characterization studies (for example, analysis of patterning efficiency), all gels were included in characterization so as to capture the overall variability in tissue patterning. Microscopy and automated image scanning Imaging of hydrogels containing live cells stained with calcein, AM or calcein red-orange, AM (Invitrogen) was performed on a Nikon Eclipse TE200 or Olympus FV1000 Multiphoton Laser Scanning Confocal Microscope. For epifluorescence images, image viewing and analysis was performed in ImageJ (NIH) and Photoshop (Adobe). For multiphoton images, z dimension between each slice was 1–2 μm. Images were stacked and merged for x–y–z extended focus images, x–z sections, and movies using Volocity 3D Image Analysis software (PerkinElmer). Automated image scanning of hydrogels containing microorganized cells was performed using a Nikon Eclipse Ti microscope equipped with an automated stage-scanning system. For studies determining patterning efficiency, hydrogels of 1.5 cm diameter containing micropatterned cells were scanned and analysed. Serial 4 × magnification images were obtained and stitched automatically using NIS Elements software (Nikon; version 3.2). Image analysis and aggregate size quantification was performed using NIS Elements software. Immunohistochemistry For immunostaining of cellular aggregates, aggregates were collected from microwells, fixed in methanol and 10% acetic acid and gently pelleted in eppendorf tubes. Aggregates were resuspended in molten histogel (Thermo Scientific), repelleted and placed on ice for histogel solidification. Histogel pellets were processed, embedded and sectioned for immunohistochemistry. Sections were stained with a primary antibody against pan-cytokeratin (1:800, Sigma) followed by secondary Alexa 488-conjugated goat-antimouse antibody (Jackson ImmunoResearch). Images were obtained using a Nikon Eclipse TE200 microscope. Tissue sections from in vivo studies were stained with primary antibodies against arginase-1 (1:400, Sigma) and/or Ter-119 (1:100, BD Pharminigen) followed by Alexa 594 or 488-conjugated donkey anti-rabbit and donkey anti-rat secondary antibodies. Biochemical assays to assess hepatocyte function Rat albumin in sampled media was quantified by enzyme-linked immunosorbant assay using a sheep anti-rat albumin antibody and rat albumin ELISA kit (Bethyl labs). In vivo implantation and assessment of engineered tissues All animal procedures were approved by The Committee for Animal Care in the Department of Comparative Medicine at Massachusetts Institute of Technology. Taconic NCr nude mice (female, 6–8 weeks old) were anesthetized using isofluorane, and engineered tissues were placed into the IP space on the day following tissue fabrication via a 1-cm incision. The incision was closed aseptically, and animal recovery from surgery was monitored. Animals were administered 0.1 mg ml −1 buprenorphine every 12 h for 3 days following surgical procedures. To enable noninvasive imaging of hepatic function and survival of engineered tissues, hepatocytes were transduced in suspension culture immediately after isolation with a lentiviral vector expressing firefly luciferase under the human albumin promoter ((pTRIP.Alb.IVSb.IRES.tagRFP-DEST, gift of Charles Rice, The Rockefeller University) before engineered tissue fabrication. For viral transduction, concentrated virus was diluted 1:5 into hepatocyte media containing HEPES buffer (20 mM; Invitrogen) and polybrene (4 μg ml −1 , Invitrogen) in six-well ultra-low-attachment plates (Corning). To aid in the establishment of intercellular junctions during viral transduction, hepatocytes were added to transduction mixture for a final concentration of 1 million hepatocytes per ml such that small clumps of ~2–5 cells formed over the course of the 5 h viral transduction (final viability after transduction ~75%). Immediately before imaging, mice were injected intraperitoneally with 250 μl of 15 mg ml −1 D -Luciferin (Caliper Life Sciences) and imaged using the IVIS Spectrum (Xenogen) system and Living Image software (Caliper Life Sciences). Upon killing, engineered tissues were retrieved, fixed in 4% paraformaldehyde, processed, embedded and sectioned for immunohistochemistry. Statistical analysis Experiments were independently repeated three times. All data in graphs are expressed as the mean±s.e./s.d. as listed in the text or figure legends. For normally distributed data, statistical significance was determined using Student’s t -test for two-way comparisons or one-way ANOVA followed by Tukey’s post-hoc test for group comparisons. Otherwise non-parametric Mann–Whitney (for two-way comparisons) or the Kruskal–Wallace test followed by Dunn’s Multiple Comparison (for group comparisons) was used. Alpha was set to 0.05 for all comparisons. How to cite this article: Stevens, K. R. et al . InVERT molding for scalable control of tissue microarchitecture. Nat. Commun. 4:1847 doi: 10.1038/ncomms2853 (2013).